Germanium avalanche receiver for low power interconnects Recent advances in silicon photonics have aided the development of on-chip communications. Power consumption, however, remains an issue in almost all integrated devices. Here, we report a 10 Gbit per second waveguide avalanche germanium photodiode under low reverse bias. The avalanche photodiode scheme requires only simple technological steps that are fully compatible with complementary metal oxide semiconductor processes and do not need nanometre accuracy and/or complex epitaxial growth schemes. An intrinsic gain higher than 20 was demonstrated under a bias voltage as low as −7 V. The Q-factor relating to the signal-to-noise ratio at 10 Gbit per second was maintained over 20 dB without the use of a trans-impedance amplifier for an input optical power lower than −26 dBm thanks to an aggressive shrinkage of the germanium multiplication region. A maximum gain over 140 was also obtained for optical powers below −35 dBm. These results pave the way for low-power-consumption on-chip communication applications. Silicon photonics have generated a growing interest for a large range of applications including optical telecommunications and on-chip optical interconnects [1] , [2] , [3] , [4] , [5] , [6] , [7] , [8] , [9] . The main challenges of silicon photonics are now power consumption and cost reductions as well as the increase in bit rate of optical integrated circuits. The cost reduction will be addressed by large scale production in 200 mm and/or 300 mm fabrication lines, whereas the consumed energy/bit and the transmission bit rate figures will only be solved by improving the devices themselves. On the receiver part, several levers exist to reduce the power consumption. The use of avalanche photodiodes (APD) could push the responsivity beyond the limit imposed by external quantum efficiency by multiplying the photogenerated carriers, leading to a reduction of the overall optical power into the photonic circuit. The reduction of the capacitance of the photodetectors also helps in reducing power consumption. Finally, a consequent amount of energy will be saved if trans-impedance amplifier (TIA) can be suppressed. Germanium photodetectors integrated in silicon waveguides have now demonstrated impressive results and have now reached characteristics close to those of their III-V semiconductor counterparts [10] , [11] , [12] , [13] , [14] . High responsivity and high speed operation have been demonstrated for these structures and Ge waveguide detectors are now considered as mature devices ready for production [15] . However, their sensitivity still remains low, about −21 dBm at 14 Gbit per second (Gbps) and bit-error-rate (BER) of 10 −12 for Ge p-i-n photodiode [16] . In most of the cases, as the photodiode dark current remains rather low (typically <1 μA), the receiver sensitivity using p-i-n photodiodes is limited by the noise of the TIA. The development of receiver-less, low capacitance photodetectors [17] , [18] , [19] (with capacitances typically of the order of ~fF or below) is thus a real challenge. Furthermore, substantial power consumption reduction could be achieved by eliminating the need for a TIA. The promising solution is to use low power and reliable avalanche photodetectors to drastically improve the sensitivity and reduce the optical power needed at given BER and bit rate, respectively. Avalanche operation of germanium-based photodiodes has been demonstrated in separate absorption charge multiplication [3] , [20] and metal semiconductor metal [4] structures. On the one hand, the first ones exhibit low multiplication noise thanks to the use of Si in the multiplication layer. However, a high bias is then needed (>−20 V). On the second hand, internal gain in metal semiconductor metal structures [4] can be achieved at low bias (<−3 V), but the associated dark currents were high (50 μA for unit gain) and degraded the sensitivity and the gain was limited. In this work we propose to use a compact p-i-n Ge photodiode biased in avalanche mode with a thin multiplication Ge layer for dead space enhanced noise reduction, for receiver-less operation at 10 Gbps. An intrinsic gain of several 10s with low signal-to-noise ratio (SNR) was demonstrated under a bias voltage as low as −7 V. 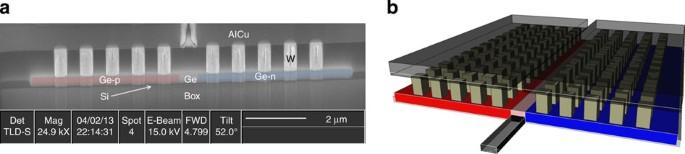Figure 1: Lateral p-i-n Ge on Si photodiode integrated at the end of a Si waveguide. (a) SEM view of the fabricated photodiode. The Ge and the Si seed layer thicknesses are around 300 and 40 nm, respectively. (b) Schematic view of the lateral p-i-n- photodiode. Standard complementary metal oxide semiconductor metallization was used with tungsten (W) plug-type contacts on Ge followed by aluminium copper (AlCu) electrodes. Design and fabrication of Ge APD Figure 1 shows a schematic view and a scanning electron microscopy image of a p-i-n diode-based Ge APD integrated in a Si waveguide. Both absorption and multiplication take place in the Ge layer. The multiplication process is initiated by electrons and holes, and both are multiplied within the intrinsic region. According to the impact ionization theory [21] , [22] , [23] , [24] , a high excess noise factor should then be obtained as electrons and holes have quite similar impact ionization coefficients in Ge [25] . However, a narrow width multiplication region (500 nm) was chosen in the design to promote a large dead space effect [23] , [26] contribution favouring an efficient reduction of the excess noise factor. Even if electrons and holes equally contribute to the noise (that is, the effective k ratio of the ionization coefficients of holes and electrons is close to unity), sensitivity can be improved without any significant dead space compared with a p-i-n photodiode operating without gain. The Ge layer is 300 nm thick and 10 μm wide and long. The intrinsic region, designed to have a width of 500 nm, was defined by the ion implantation of n-type and p-type regions. The narrow intrinsic Ge region ensures the presence of a high electric field inside the intrinsic region over the full depth. Efficient butt-coupling of light is obtained by the direct connection of Si waveguide and the Ge absorption layer. The input Si waveguide was designed to be single mode at λ =1,550 nm with TE polarization. Resulting width and height are 500 and 220 nm, respectively. A 10-μm long Ge layer was selectively grown by reduced pressure–chemical vapour deposition in an etched Si recess at the end of the waveguide (see Methods), yielding high absorption efficiency with a small device capacitance. The back-end-of the-line processing consisted in standard complementary metal oxide semiconductor metallization with tungsten (W) plug-type contacts on Ge followed by aluminium copper (AlCu) electrodes. Figure 1: Lateral p-i-n Ge on Si photodiode integrated at the end of a Si waveguide. ( a ) SEM view of the fabricated photodiode. The Ge and the Si seed layer thicknesses are around 300 and 40 nm, respectively. ( b ) Schematic view of the lateral p-i-n- photodiode. Standard complementary metal oxide semiconductor metallization was used with tungsten (W) plug-type contacts on Ge followed by aluminium copper (AlCu) electrodes. Full size image The room temperature characteristics for current and gain versus applied bias are shown in Fig. 2 . The dark current is about 18 nA under −1 V bias and increases up to 610 μA under −7 V. The dark current generation in such Ge on Si photodiodes has a strong electric field dependence. Since tunnelling is very important at high electric fields in Ge, notably because of its low bandgap energy, the dark current already reaches high levels before that multiplication occurs. When the avalanche gain starts to rise, both impact ionization and tunnelling were competing. It is usually supposed, when calculating the noise power and/or the sensitivity, that the dark current is constant with the electric field for a unit gain. This assumption is correct for materials in which tunnelling rate is small and bandgap energy rather high. It may however introduce, notably for Ge, quite a large sensitivity estimation error. In receivers based on p-i-n photodiodes operating without gain but with a TIA, the sensitivity is most often limited by the TIA noise unless the PD dark current is of the order of the μA. Multiplication noise is by contrast the main noise limitation when the PD is operated in avalanche mode. In Ge on Si photodiodes, the Ge layer is grown by heteroepitaxy on a lattice-mismatched substrate. A large number of dislocations, which act as generation centres are then present in the Ge layer. By adjusting the growing conditions and post-epitaxial annealing steps, the Ge crystalline quality can still be optimized to reduce the threading dislocation density, thereby reducing the dark current (see Methods). The low-field dark currents measured here are among the best reported so far for lateral p-i-n Ge on Si photodiodes integrated at the end of waveguides with an ion implantation scheme. A further decrease of the dark current may be possible with other growth techniques and/or integration strategies. However, the aim here was to develop devices that can be easily integrated with other photonic devices such as modulators and passives devices, within the same fabrication flow and processes. 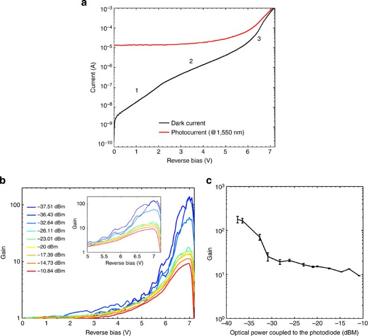Figure 2: Current–voltage and gain–voltage characteristics of the Ge p-i-n photodiode. (a) Dark and photocurrent measurements at room temperature. A 1,550 nm wavelength laser source was used to generate photocurrent. The power coupled to the photodiode was estimated to be around 33.6 μW. (b) Gain versus applied reverse bias for several optical powers coupled to the photodiode at 1,550 nm wavelength. Gain characteristics were extracted from the photocurrent and dark current measurements (c) Maximum gain at a wavelength of 1,550 nm as a function of the optical power coupled to the photodiode. Error bars correspond to the gain variance calculated from gain fluctuations. Figure 2: Current–voltage and gain–voltage characteristics of the Ge p-i-n photodiode. ( a ) Dark and photocurrent measurements at room temperature. A 1,550 nm wavelength laser source was used to generate photocurrent. The power coupled to the photodiode was estimated to be around 33.6 μW. ( b ) Gain versus applied reverse bias for several optical powers coupled to the photodiode at 1,550 nm wavelength. Gain characteristics were extracted from the photocurrent and dark current measurements ( c ) Maximum gain at a wavelength of 1,550 nm as a function of the optical power coupled to the photodiode. Error bars correspond to the gain variance calculated from gain fluctuations. Full size image Dark current and gain measurements The dark current characteristic presented in Fig. 2a exhibits three regimes which are explained by different contributions. The first region (noted 1 in Fig. 2a ) corresponds to bulk generation due to Shockley–Read–Hall and trap-assisted tunnelling at low electric fields, up to ~2.2 V. An increase of the band-to-band tunnelling contribution, which dominates carrier generation at high electric fields, occurs in the second region (noted 2 in Fig. 2a ). Region 2 ends when the avalanche gain starts to rise significantly (that is, close to 5 V). 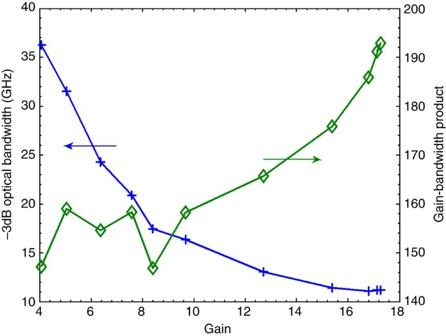Figure 3: −3 dB optical bandwidth versus gain. Optical bandwidth was measured atλ=1,550 nm with −19 dBm of optical power coupled to the photodiode. The different gain values correspond to different applied reverse biases. At a gain of ~17, the photodiode −3 dB bandwidth reaches 11 GHz. Gain bandwidth is also represented with ordinate axis on the right side. This has been experimentally verified by temperature measurements of the dark current function of the applied bias and activation energy extraction ( Supplementary Data and Supplementary Figure 3 ). At even higher fields (region 3), the generation is dominated by the multiplication process, giving rise to a more abrupt evolution of the carrier’s generation. The photocurrent shown in Fig. 2a was measured at a wavelength of 1,550 nm with a −14.73 dBm optical power coupled to the photodiode. Thus, nominal responsivity (at unity gain) was measured to be 0.4 A W −1 . This value is below its theoretical limit of 1.25 A W −1 , and can be explained in terms of generation efficiency. From two-dimensional ion implantation simulations, calibrated with secondary ion mass spectroscopy, we demonstrated that the intrinsic region was reduced due to the diffusion and lateral channelling of the dopants. By fitting the current–voltage characteristic with a p-i-n junction analytical model, including breakdown, the extracted width of the intrinsic region was found to be around 280 nm. In addition, we have measured several devices with longer and wider intrinsic regions (for example, 50 μm long and 1 μm wide). A 1.2 A W −1 responsivity was then obtained, showing that the collection efficiency is very good in our Si/Ge heterostructures. The responsivity reduction in our narrow intrinsic Ge region avalanche devices is thus mainly imputable to a generation efficiency loss (absorption in the doped regions nearby and an absorption length which is not high enough). The gain dependency on the optical power has been further investigated. As expected, the lower the incoming power, the higher the gain. Figure 2b shows the measured gain as a function of the reverse bias for different input optical powers at λ =1,550 nm. For very low optical power, the photocurrent is close to the dark current in the gain regime. Dark current fluctuations then increase the gain determination uncertainty, resulting in the gain fluctuations seen in Fig. 2 . The gain reaches a maximum value before decreasing due to the carrier density inside the junction. As the carriers’ density increases, both phonon scattering and space charge effect occur, lowering the gain. The strong dependence of the maximum static gain as a function of the optical power is shown in Fig. 2c . As expected, the gain increases when the input optical power decreases. A gain >140 is reached for optical powers below −35 dBm. The capacitance was also measured as a function of the reverse bias using a calibrated impedance meter ( Supplementary Fig. 1 ) over a full 200-mm wafer. The low bias capacitance (typically <2 V of reverse bias) was voltage dependent, indicating that the intrinsic region was not fully depleted. Indeed, a variation from 18 fF to 5 fF was obtained from 0 V to −2 V. Below −2 V, the capacitance saturated at values <5 fF, with nearly 4 fF under −3 V reverse bias. According to these capacitance value, the RC (resistance × capacitance) limited bandwidth remains over 35 GHz under gain regime. 10 Gbps measurements under gain regime The optical bandwidth was measured using a network analyzer and a 1,550 nm wavelength modulated laser source (see Methods). Figure 3 shows the −3 dB optical bandwidth at λ =1,550 nm of a p-i-n photodiode as a function of the gain for a −19 dBm optical power. When the photodiode is operated with unity gain, the maximum bandwidth is >40 GHz. As the gain increases, the bandwidth decreases as the carrier multiplication time then increases. Both holes and electrons contribute to impact ionization in germanium as their ionization coefficients are rather similar. The multiplication time therefore increases compared with a material where only one type of carrier impact ionizes (that is, Si) [27] . Hence, the bandwidth drops, as it is dominated by the multiplication time. At a gain of 17, the measured photodiode bandwidth yet remains about 11GHz, allowing a 10 Gbps operation. The gain-bandwidth product is then >190 GHz. Figure 3: −3 dB optical bandwidth versus gain. Optical bandwidth was measured at λ =1,550 nm with −19 dBm of optical power coupled to the photodiode. The different gain values correspond to different applied reverse biases. At a gain of ~17, the photodiode −3 dB bandwidth reaches 11 GHz. Gain bandwidth is also represented with ordinate axis on the right side. Full size image To further investigate the dynamic properties of APD, eye diagram measurements were performed. No TIA was used. The photodiode was directly connected to the sampling oscilloscope using a bias tee and radio-frequency probes (see Methods). As a reference, an eye diagram was measured with a −4.26 dBm optical power coupled to the photodiode, biased under −2 V ( Fig. 4a ). Assuming a Gaussian noise distribution, the Q -factor was calculated from the measured eye diagram (see Methods). A Q -factor of 8.11 and an extinction ratio of 12.6 dB were extracted from those measurements. 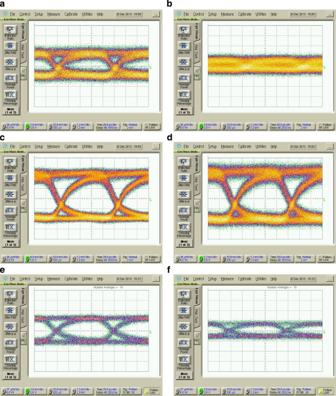Figure 4: 10 Gbps eye diagrams measured at a wavelength of 1,550 nm. (a) Under 2 V reverse bias with −11.25 dBm optical power coupled to the APD (unity gain), (b) under 2 V reverse bias with −14.6 dBm optical power coupled to the APD, (c) under 7 V reverse bias with −11.25 dBm optical power with a gain of 10, (d) under 7 V reverse bias with −14.6 dBm optical power with a gain of 11, (e) under 7 V reverse bias with −23 dBm optical power with a gain of 15 and (f) under 7 V reverse bias with −26 dBm optical power with a gain of 20. Figure 4 shows 10 Gbps eyes diagrams for several optical input powers and reverse biases. Figure 4a,c show eye diagrams, respectively, at unity gain (under 2 V of reverse bias) and at gain of 10 (under a 7 V reverse bias) for a −11.25 dBm optical power coupled to the photodiode. The extracted Q -factor was equal to 4.2 without any gain and improved to 8.12 with a gain of 10, respectively. According to the BER definition, such a Q -factor of 8.12 corresponds to a BER of 2.33.10 −16 . The extinction ratio is also improved from 4.7 dB without any gain to 9.28 dB with a gain of 10. By reducing the optical power by a factor of 5, we were able to recover the same Q -factor with a gain of only 10, hence the same SNR. By further reducing the optical power to −14.6 dBm, the eye diagram without any gain closes itself (−2 V bias), as seen in Fig. 4b . However when the photodiode is biased in avalanche mode, here at −7 V (which corresponded to a gain of 11), the eye diagram is definitely opened, as seen in Fig. 4d . The calculated Q -factor in this case is 7.06 and the extinction ratio reaches 12.75 dB. As the optical power goes down, the gain increases at a fixed bias of −7 V. For −23 and −26 dBm, the measured gain values are 15 and 20, respectively. The corresponding eye diagrams are shown in Fig. 4e,f , respectively. The eye diagrams are still well opened with extinction ratio of 5.2 and 2.77 dB and Q -factors of 6.94 and 5.09 for input powers of −23 dBm and −26 dBm. Such a Q -factor at −26 dBm corresponds to a BER of 1.8 × 10 −7 . It means that for a −26 dBm optical power, a BER of 1.8 × 10 −7 is achievable at 10 Gbps without any amplification stage. Figure 4: 10 Gbps eye diagrams measured at a wavelength of 1,550 nm. ( a ) Under 2 V reverse bias with −11.25 dBm optical power coupled to the APD (unity gain), ( b ) under 2 V reverse bias with −14.6 dBm optical power coupled to the APD, ( c ) under 7 V reverse bias with −11.25 dBm optical power with a gain of 10, ( d ) under 7 V reverse bias with −14.6 dBm optical power with a gain of 11, ( e ) under 7 V reverse bias with −23 dBm optical power with a gain of 15 and ( f ) under 7 V reverse bias with −26 dBm optical power with a gain of 20. Full size image As the optical power is kept at −11.25 dBm, the Q -factor nearly doubles by increasing the gain from unity to 10. According to the McIntyre’s theory [24] , the shot noise should also have then increased since the ionization coefficient ratio is close to unity in Ge. The excess noise factor should therefore have increased almost linearly with the gain. This suggests that the gain variance is small, hence it begins almost deterministic. This can be explained by looking at the excess noise factor when the dead space is not negligible anymore [28] . The dead space is indeed defined as d = E i / qF , where E i is the ionization threshold energy, q the elementary charge and F the electric field strength. Using E i values from Okuto and Crowell [29] and supposing that the electric field strength is 200 kV cm −1 (from our own analytic calculation under −7 V bias), the dead space is estimated to be around 50 nm, which is not negligible compared with the 280-nm wide multiplication region. The experimental excess noise has been determined from eye diagram noise measurements with a −11.25 dBm optical power. At both M =1 and M =10, the experimental excess noise was found to be equal to 5.24 ( Supplementary Discussion ). For Ge, as both electrons and holes have similar ionization coefficients, the ratio is expected to be ~0.9. Using McIntyre [24] expression for the excess noise factor led to an effective ratio of ionization coefficient keff~0.4. This value confirms the observed noise reduction, which is attributed to the dead space effect. We demonstrated the great potential of integrated p-i-n Ge photodiodes in silicon photonics circuits for avalanche operation under low bias voltages. Such APD enables an easy integration in CMOS process flows. Ten Gbit per second open eye diagrams at several optical powers and significant gains were obtained without the use of an amplification stage, offering the possibility of using Ge avalanche photodiodes as receiver-less photodiodes for on-chip optical communication applications. The eye diagrams Q -factor were maintained >14dB even at low optical powers of −26 dBm, and responsivity reached 8 A W −1 . The noise reduction enhancement by dead space was evidenced as thin multiplication regions were designed. The future integration of such photodiodes with low noise TIA and equalizer should lead to very high sensitivity receivers for optical communication applications requiring low power consumption. Moreover, we were able to achieve a gain >140, which is among the highest reported so far for Ge APDs, albeit with much more complex integration schemes. This demonstration may enable the development of new applications including secure quantum key distribution [30] , which requires photon counting receivers, as well as on-chip optical clocking [18] . Device fabrication All devices were fabricated on 200-mm silicon-on-insulator wafers, with 2 μm buried oxide and 220-nm Si layers. Waveguides and grating couplers were first fabricated, resulting in 220 × 500 nm single-mode waveguides. A 10 × 10 μm cavity was partially etched at the end of the waveguide; the remaining Si layer served as a seed layer for the Ge heteroepitaxy. A ‘HF-Last’ wet cleaning followed by an in-situ H 2 bake at 850 °C, 20 Torr (in a 200 mm Epi Centura reduced pressure–chemical vapour deposition tool from Applied Materials) was used to prepare the surface of the Si windows before Ge selective epitaxy. A thin Ge layer (~40 nm) was then grown at 450 °C, 100 Torr, followed by a more than 1 micron thick Ge layer at 750 °C, 20 Torr. A short thermal cycling under H 2 (between 750 and 875 °C) was used afterwards to reduce the threading dislocations density [31] ( Supplementary Fig. 2 ). The significant loading effects (that is, growth rate increases) inherent to such patterned wafers were accounted for thanks to (i) a downscaling of the GeH 4 mass-flow (the gaseous precursor of Ge) and (ii) the use of significantly shorter growth times than on blanket wafers. The excess Ge overflowing the cavity was removed by chemical mechanical polishing, with a 300-nm thick remaining thickness. To form the p-i-n diode, the Ge was doped by ion implantation of boron and phosphorous and the dopants activated by rapid thermal annealing. Ti/TiN/W plugs were formed to contact the Ge layer, followed by AlCu deposition and patterning for pads definition. Gain determination The gain was extracted from the I – V measurements. The photocurrent did not show any voltage dependency before multiplication occurred. The 0 V photocurrent served as the reference photocurrent for gain determination. The gain corresponds to the ratio of the photocurrent (that is, the total current minus the dark current) by the reference photocurrent. Capacitance measurements To determine the capacitance of the fabricated photodiodes, an LCR meter was used. Prior calibrations ensured precise measurements in the fF range. The capacitances were measured at 1 MHz, function of the applied reverse bias, from 0 to −3 V, by steps of 0.1 V. The photodiode was biased using a Keithley Source Measurement Unit. Bandwidth measurements Bandwidth measurements were performed with a 50-GHz HP Agilent 86030A Lightwave Component Analyzer at 1,550 nm. The photodiode were biased through a bias tee by a Keithley Source Measurement Unit. Prior calibrations of the radio-frequency path were done to get rid of the cables and probe contributions. Optical −3 dB bandwidth was extracted as a function of the applied bias. Eye diagram measurements Eye diagrams were measured using commercial lithium-niobate modulator. A 2 7 −1 pseudo-random binary sequence NRZ optical bit stream was then generated at a wavelength of 1.55 μm and coupled into Ge APD using grating coupler. Eye diagrams were recorded using 50 GHz sampling oscilloscope from Agilent. Parameter determination The Q-Factor is extracted from the eye diagram measurements following the definition given by Personick [32] : . Where s 1 and s 0 are the signal amplitude mean values for a 1 and a 0 respectively, and σ 1 and σ 0 the associated standard deviation. The BER can then be obtained assuming Gaussian noise distribution: . The Q -factor is an evaluation of the SNR at the output of the photodiode. How to cite this article: Virot, L. et al . Germanium avalanche receiver for low power interconnects. Nat. Commun. 5:4957 doi: 10.1038/ncomms5957 (2014).